Size and mechanics effects in surface-induced melting of nanoparticles Various melting-related phenomena (like surface melting, size dependence of melting temperature, melting of few nm-size particles and overheating at a very fast heating rate) are of great fundamental and applied interest, although the corresponding theory is still lacking. Here we develop an advanced phase-field theory of melting coupled to mechanics, which resolves numerous existing contradictions and allowed us to reveal exciting features of melting problems. The necessity of introducing an unexpected concept, namely, coherent solid–melt interface with uniaxial transformation strain, is demonstrated. A crossover in temperature dependence of interface energy for radii below 20 nm is found. Surface-induced premelting and barrierless melt nucleation for nanoparticles down to 1 nm radius is studied, and the importance of advanced mechanics is demonstrated. Our model describes well experimental data on the width of the molten layer versus temperature for the Al plane surface and on melting temperature versus particle radius. Numerous melting-related phenomena represent fundamental material problems and are currently under intense experimental and theoretical study. They include surface premelting and melting below the thermodynamic melting temperature θ e , caused by reduction in surface energy and leading to appearance of a molten, nanometer-thick layer [1] , [2] ; reduction in melting temperature θ m with reduction of the particle radius R down to nanoscale [3] , [4] ; melting of particles with radii comparable to and smaller than the equilibrium solid–liquid interface width δ e , which is a few nm [3] , [5] ; and overheating above θ e during very fast heating [6] , [7] . All of these phenomena allow one to determine the properties of solid and liquid deeply in the region of their metastability and even complete instability (that is, above the solid instability temperature θ i or below the melt instability temperature θ c , see Supplementary Fig. S1 ), and to study intermediate states, various scale effects and non-equilibrium thermodynamic and kinetic properties. These studies also have important applied aspects, for example, for combustion of Al nanoparticles [8] , which are the most known representatives of nanoenergetic materials. However, a consistent theoretical framework for the description of the above phenomena is lacking. The sharp-interface approach [9] (SIA) is not justified for the above problems. Although there are important molecular dynamics (MD) studies [5] , [6] , [10] , we focus on the continuum phase-field approach (PFA), which allows consideration of larger spatial and time scales and operates explicitly with thermodynamic and kinetic parameters determined at the macroscale (see Supplementary Discussion ). When mechanics is taken into account, a basic problem of the description of finite-width, solid–liquid interface appears. Traditionally, solids and liquids are described in completely different continuum mechanical frameworks (for example, solids are described in undeformed states, whereas liquids are described in a deformed state), which sophisticates the description of intermediate state. Some works consider solid as a very viscous liquid [13] , that is, neglect elastic shear modulus μ . Such a liquid–liquid interface is incoherent and does not generate internal elastic stresses, similar to sharp interface ( Fig. 1 ). Alternatively [14] , solid–melt interface is considered as a coherent interface ( Fig. 1 ), in which shear modulus varies from that for solid to zero, and this results in generation of internal elastic stresses at the interface. When particle size is comparable to or smaller than the interface width, a coherent interface is the only reasonable choice. Although this model is supposed to be more precise, the surface tension in it is not consistent with sharp-interface limit, even if μ =0. Also, even for liquid–liquid interface, expression for surface tension in PFA differs by a hydrostatic pressure from that in SIA [11] , [12] , [13] . This is a fundamental thermodynamic inconsistency, which is especially important for nanoscale interface radii. 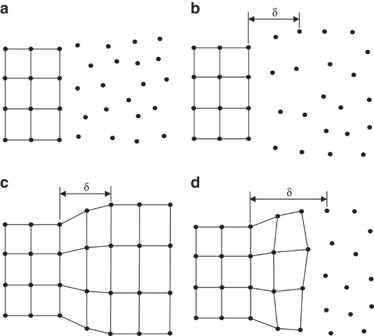Figure 1: Different types of interfaces between solid and molten phases. (a) Traditional sharp incoherent solid–melt interface, which does not generate internal elastic stresses. (b) Incoherent, finite-width, solid–melt interface with zero shear modulusμ=0 that does not generate internal elastic stresses. (c) Coherent finite-width interface between two solid phases. Continuity of crystal lattice across the interface along with a change in the size of one of the lattices during transformation (due to transformation strain tensorɛt) generates internal elastic stresses. (d) Coherent, finite-width, solid–melt interface with non-zero shear modulusμ≠0 that generates internal elastic stresses. Figure 1: Different types of interfaces between solid and molten phases. ( a ) Traditional sharp incoherent solid–melt interface, which does not generate internal elastic stresses. ( b ) Incoherent, finite-width, solid–melt interface with zero shear modulus μ =0 that does not generate internal elastic stresses. ( c ) Coherent finite-width interface between two solid phases. Continuity of crystal lattice across the interface along with a change in the size of one of the lattices during transformation (due to transformation strain tensor ɛ t ) generates internal elastic stresses. ( d ) Coherent, finite-width, solid–melt interface with non-zero shear modulus μ ≠0 that generates internal elastic stresses. Full size image Surface premelting and melting were studied using PFA [15] , [16] , [17] without involving mechanics. However, the employed equation for surface energy, γ ( η )= a + bη 2 , did not allow a homogeneous solution for solid ( η =1) ( Fig. 2 ), exhibiting a surface disordered structure even below melt instability temperature θ c , when the energy minimum corresponding to melt does not exist. Such an inconsistency also exhibits itself in unphysical regions in the phase diagram [15] . 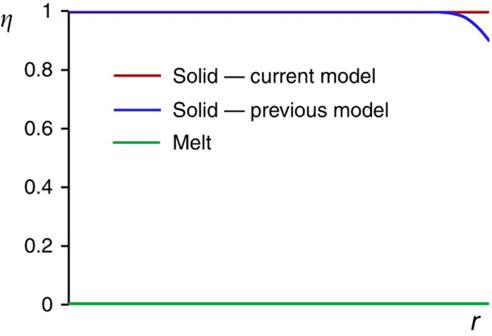Figure 2: Stationary solutions for Ginzburg–Landau equation with different models for surface energy. Previous models15,16,17(blue line) did not allow a homogeneous solution for the solid (η=1), exhibiting a surface disordered structure at any temperature. Our model equation (8) (red line) is developed using the condition that it allows a homogeneous solution for the solid. The green line represents melt (η=0). Figure 2: Stationary solutions for Ginzburg–Landau equation with different models for surface energy. Previous models [15] , [16] , [17] (blue line) did not allow a homogeneous solution for the solid ( η =1), exhibiting a surface disordered structure at any temperature. Our model equation (8) (red line) is developed using the condition that it allows a homogeneous solution for the solid. The green line represents melt ( η =0). Full size image The goal of this paper is to develop a unified PFA coupled to mechanics and reveal the non-trivial features of the above melt-related phenomena. Thus, a model with coherent solid–melt interface is developed (see Fig. 1 ), in which shear modulus μ varies from that for solid to zero, and this results in generation of internal elastic stresses at the interface. Thermodynamic potential in this model results in surface-tension stresses consistent with the SIA, in contrast to known models with incoherent interface (for which μ =0) [11] , [12] , [13] and coherent interface [14] . Also, the necessity of introducing a non-spherical transformation strain, which, in addition to volumetric expansion during melting, describes change in shape, is demonstrated. Our model resolves fundamental thermodynamic inconsistency and includes more advanced mechanics, which is especially important for nanoparticles. Also, a model for surface energy that varies during melting is developed, which resolves the aforementioned non-physical effects in existing models [15] , [16] , [17] and adds mechanics to them. It is demonstrated that our model describes well experimental data on the width of the molten layer versus temperature for the Al plane surface, and then it is applied to surface-induced premelting and barrierless melt nucleation for nanoparticles. It also describes well experimental data on θ m versus R , even better than MD simulations [5] . Then, non-equilibrium and small-scale regimes were treated, that is, interface profile, width, energy and velocity have been determined and analysed versus R , interface position r i , and large overheating and heating rates ħ . Thus, the derived analytical expression for interface velocity v describes well simulation results well outside an expected range, namely, even for θ > θ i , ħ up to 10 13 K s −1 , and r i ≥2 δ e . It also describes well the effect of large compressive and tensile pressure. Homogeneous melt nucleation competes for ħ =10 13 K s −1 with interface propagation. For R =1 and 3 nm, premelting occurs in the entire particle rather than at the surface only. Allowing for mechanics increases the melting temperature by 70 K for R =1 nm particle due to pressure induced by surface tension. For R ≤1.5 nm, θ m < θ c , that is, the particle melts more than 200 K below θ e , while there is no local energy minimum corresponding to melt. While for a liquid–liquid interface our calculations reproduce the Laplace relationship for jump in radial stresses Δ σ r , for coherent solid–melt interface, Δ σ r does not follow the Laplace relationship and even may possess the opposite sign, causing tension in the solid core instead of compression. Interface energy varies in a non-trivial way for r i ≤4 δ e ≃ 12 nm with decreasing r i , increasing for θ > θ e and decreasing for θ < θ e ; this is opposite to the behaviour for r i >12 nm. Theory We designate contractions of tensors A ={ A ij } and B ={ B ji } over one and two indices as A · B ={ A ij B jk } and A : B = A ij B ji , respectively. The subscript * means symmetrization; the subscripts or superscripts e , θ and t are for elastic, thermal and transformational contributions to strain and energy; I is the unit tensor; Δ A = A s − A m for any property A , with subscripts s and m denoting solid and melt, respectively; and are the gradient operators in the undeformed and deformed states; and ⊗ designates a dyadic product. To develop a unified approach to solid and liquid, we will consider liquid as the limit case of isotropic viscoelastic solid with μ =0. For simplicity, viscosity is neglected, isothermal processes are considered and shear strain is small. However, even if volumetric strain ɛ 0 is small, in order to reproduce surface tension one has to use fully large-strain formulation (see below). We will modify our recently developed theory of martensitic transformations in solids [18] , [19] to describe melting. The Helmholtz free energy per unit undeformed volume of solid ψ = ψ ( ɛ , η , η , θ ), in which ɛ is the strain tensor and η is the order parameter that varies from 1 in solid to 0 in melt. Using an irreversible thermodynamic procedure based on the application of the first and second laws of thermodynamics to the system with energy depending on the gradient of the order parameter (see ref. 12 and references in it) and assuming linear relation between thermodynamic force and flux, one obtains expression for the stress tensor σ and the Ginzburg–Landau (GL) equation in which ρ 0 and ρ are the mass densities in the non-deformed and deformed states, χ is the kinetic coefficient, and ɛ =const while evaluating ∂ψ / ∂η . The kinematics relationship between displacement u and strain ɛ =1/3 ɛ 0 I + e , decomposition of ɛ and the equilibrium equation are given by in which e is the deviatoric strain. Energies and strains are defined as follows: Here K is the bulk modulus, β and α are the gradient energy and linear thermal expansion coefficients, H is the heat of fusion, is the double-well energy, and is the transformation strain that transforms the elemental volume of solid to melt under σ =0. While for martensitic phase transformations is a tensor connecting two crystal lattices, for melting it is always pure volumetric strain, [9] , [11] , [12] , [13] , [14] . We will show that the usual assumption causes very high internal stresses and elastic energy within the interface, which suppresses melt nucleation and contradicts with the experiment. Development of a complete theory for is not a goal of this paper, but we consider an alternative expression for uniaxial , in which is the unit normal to the interface. In this case, the component of transformation strain along the interface is absent, which minimizes internal stresses and their energy. Then equation (1) looks like in which σ e and σ st are the elastic stress and surface tension, σ e = p e for volumetric transformation strain and σ e = k · σ e · k for uniaxial transformation strain. For a phase-equilibrium condition in the stress-free case, (ref. 20 ), and we have σ st = β | η | 2 ( I − k ⊗ k ), that is, it represents two equal normal stresses along the interface. Thus, σ st is consistent with the SIA, unlike previous approaches [11] , [12] , [13] , [14] , which resolves a long-standing problem in PFA for melting. In contrast to previous works on melting and other transformations in solids [14] , [18] , the gradient operator with respect to the deformed state was used, and the finite-strain factor J was included in the proper places. Although use of is natural for liquids [11] , [12] , [13] , this is not the case for solids. One of the unexpected points is that even for small strains, one cannot assume that J ≃ 1 and , because this leads to zero surface tension. The same thermodynamic procedure [19] that led to equation (1) also results in the boundary conditions in which n is the unit normal to the boundary, σ n is the normal to interface stress, 1/ R is the mean curvature and is the external pressure. Equation (8) represents a generalization for the 3-D case and coupling with mechanics of known condition [15] , [16] . We require the following properties of the surface energy: γ (0)= γ l ; γ (1)= γ s ; . The last equation guarantees that homogeneous melt ( η =0) and solid ( η =1) satisfy equation (8) and removes contradiction in the known papers [15] , [16] (see Fig. 2 ). These properties are met for polynomial γ ( η )= γ l +Δ γ (a η 2 +(4−2a) η 3 +( a −3) η 4 ) of the lowest degree with a parameter a . One can demonstrate that a criterion of barrierless surface-induced melt nucleation is consistent with a sharp-interface condition, Δ γ > γ s−l , when a =3. Then γ ( η )= γ l +Δ γφ ( η ). If surface energy does not change during melting, then γ =const and equation (8) reduces to traditional boundary condition η · n =0. We focus on Al nanoparticles; material parameters are given in Supplementary Discussion . In particular, θ e =933.67 K, θ c =0.8 θ e =746.9 K and θ i =1.2 θ e =1120.4 K, δ e =2.97 nm. Note that all material parameters have been obtained for a macroscopic sample with no fitting parameters left. None of our developments (coherent interface with uniaxial transformation strain, expressions for free energy that result in correct expression for surface tension, and expression for surface energy) requires additional material parameters. First, homogeneous heating of particles of radius R was considered and stationary solutions were found for each temperature. The thickness h of pre-molten and completely molten surface layer (determined by an interphase radius r i , that is, by point with η =0.5) have been plotted versus θ e − θ ( Fig. 3 ). At melting temperature, θ m , the stationary, two-phase solution ceases to exist and interface propagates to the centre. 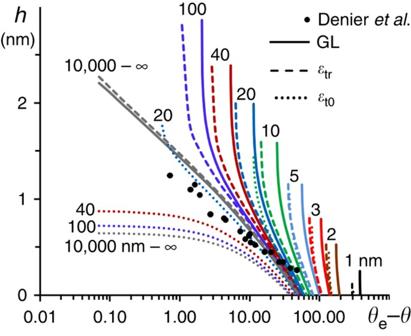Figure 3: Thickness of molten surface layer versus temperature for different particle radii. Each colour represents a particle radius shown in nm near the curves. Solid lines are results of the GL model without mechanics. Dotted and dashed lines are obtained for coupled GL and mechanics model with volumetric and uniaxial transformation strains, respectively. Black dots are experimental data1obtained using medium-energy ion scattering. Experimental points for a plane surface are close to the calculations for infinite radius for GL and coupled models with uniaxial transformation strain. All curves, excluding those interrupted at 0.1 K, are ended at the melting temperature. Figure 3: Thickness of molten surface layer versus temperature for different particle radii. Each colour represents a particle radius shown in nm near the curves. Solid lines are results of the GL model without mechanics. Dotted and dashed lines are obtained for coupled GL and mechanics model with volumetric and uniaxial transformation strains, respectively. Black dots are experimental data [1] obtained using medium-energy ion scattering. Experimental points for a plane surface are close to the calculations for infinite radius for GL and coupled models with uniaxial transformation strain. All curves, excluding those interrupted at 0.1 K, are ended at the melting temperature. 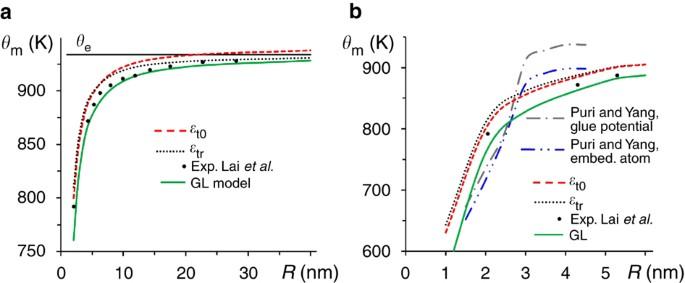Figure 4: Melting temperature of Al versus particle radius. (a) Curves are calculated using three models: GL equations only (GL, green line), GL equation coupled to mechanics with volumetric (ɛt0) (red line) and uniaxial (ɛtr) (black dotted line) transformation strain. Dots are experimental data from Laiet al.3obtained using thin-film differential scanning calorimetry. The horizontal line is the equilibrium temperature (the same curve designations are used inb). (b) Molecular dynamics results are added for particles with radii in the 1–6 nm range. Gray and blue lines are MD results5using glue and embedded atom potentials, respectively. Full size image Size dependence of melting temperature In Figure 4 , the lowest curve is for GL equation only, that is, for neglected mechanics. Below radius R *=6.12 nm, results for volumetric ɛ t give slightly lower θ m and are closer to the experimental points, whereas for R > R * results for uniaxial ɛ t are much lower. For R >21.2 nm and volumetric ɛ t , θ m > θ e . This is in contrast to the experiments for flat interface, for which θ m = θ e . That is why uniaxial transformation strain was used, in contrast to known models [11] , [12] , [13] . For neglected mechanics and for uniaxial ɛ t , melting temperature tends to θ e for infinite radius. Experimental points are between curves with neglected mechanics and for uniaxial ɛ t for R > R * and for volumetric ɛ t for R < R *. Coupling with mechanics for 2–3 nm particles increases the melting temperature by 30–40 K (see also Fig. 5 ) and makes it closer to the experiments. Surprisingly, our results are in better correspondence with experiments than known MD approaches ( Fig. 4b ). Thus, we can conclude that the model of coherent solid–melt interface has good potential for the description of experiments; traditional volumetric ɛ t is not adequate for large particles, that is, there is interface restructuring, driven by the internal stress relaxation, and a thermodynamic and kinetic theory for e t should be developed. Figure 4: Melting temperature of Al versus particle radius. ( a ) Curves are calculated using three models: GL equations only (GL, green line), GL equation coupled to mechanics with volumetric ( ɛ t0 ) (red line) and uniaxial ( ɛ tr ) (black dotted line) transformation strain. Dots are experimental data from Lai et al . [3] obtained using thin-film differential scanning calorimetry. The horizontal line is the equilibrium temperature (the same curve designations are used in b ). ( b ) Molecular dynamics results are added for particles with radii in the 1–6 nm range. Gray and blue lines are MD results [5] using glue and embedded atom potentials, respectively. 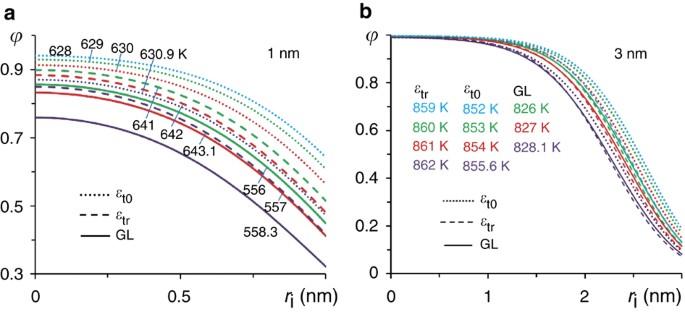Figure 5: Stationary interface profilesφ(η) for Al particles for different temperatures. (a)R=1 nm; (b)R=3 nm. Solid lines are the results obtained with the GL model. Dotted and dashed lines are obtained using coupled GL and mechanics models with volumetric and uniaxial transformation strains, respectively. Different temperatures are considered for each model, which are designated on the graphs. The lowest curve for each model corresponds to the melting temperature. Full size image Figure 5: Stationary interface profiles φ ( η ) for Al particles for different temperatures. ( a ) R =1 nm; ( b ) R =3 nm. Solid lines are the results obtained with the GL model. Dotted and dashed lines are obtained using coupled GL and mechanics models with volumetric and uniaxial transformation strains, respectively. Different temperatures are considered for each model, which are designated on the graphs. The lowest curve for each model corresponds to the melting temperature. Full size image Surface premelting and melting As shown in Figure 3 , for a plane interface ( R →∞), plots for thickness of the molten layer versus θ for GL and uniaxial ɛ t almost coincide and are very close to experimental points, which justifies the validity of our model for surface energy. Results for volumetric ɛ t are inconsistent with experiments. For nanoparticles, h ( θ ) plots consist of two parts: an almost straight line with small slope at high temperature with transition to an almost vertical line for temperatures close to θ m . The maximum thickness of the molten layer is very close for the GL model and the model with uniaxial ɛ t . Although curves for these models look also close, for some temperatures the difference in thickness is a factor of 2 or larger. For R ≤5 nm, curves for volumetric and uniaxial ɛ t are very close. Stationary distributions of interface profiles φ ( η ) (note that φ ( η ) rather than η describes the variation of all properties, see equation (1)) in particles of R =1 and 3 nm are presented in Figure 5 . For all cases, the complete liquid phase ( η =0) is not reached. For 1 and 3 nm, stationary premelting (that is, φ ( η )<1) occurs in the entire particle rather than at the surface only. Allowing for mechanics increases the melting temperature by 70 K for the R =1 nm particle, mostly due to pressure induced by surface tension. Note that for R <1.5 nm, one has θ m < θ c , that is, the particle melts even when bulk melt is unstable. 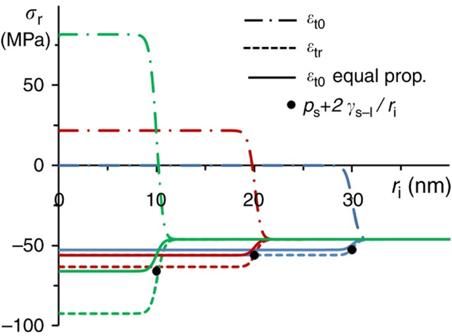Figure 6: Distribution of radial stresses for three interface positions. The blue line corresponds to the interface radius at 30 nm, the red at 20 nm, and the green at 10 nm. Distributions are calculated atθeusing models with volumetric (ɛt0) (dotted line) and uniaxial (ɛtr) (dashed line) transformation strains, as well as with equal thermoelastic properties of solid and melt (solid line), that is, for liquid–liquid transformation. Dots designate pressures in meltps+2γs−l/ribased on the Laplace equation that coincides with results of calculations for equal thermoelastic properties of the solid and melt. Surface tension Distributions of radial stresses along r are shown in Figure 6 . When internal elastic stresses can be neglected (for equal thermoelastic properties of phases and μ =0, that is, for liquid–liquid transformation, or for ɛ t =0), our calculations at θ e reproduce the Laplace relationship for jump in radial stresses Δ σ r =−2 γ s − l / r i within an error of 0.14% for r i >11 nm and 1.03% at r i =5 nm. For actual solid-melt properties and volumetric ɛ t , Δ σ r does not follow the Laplace relationship and even possesses the opposite sign, causing tension in the solid core ( Fig. 6 ). For uniaxial ɛ t , Δ σ r =− k 2 γ s−l / r i with k >1. Figure 6: Distribution of radial stresses for three interface positions. The blue line corresponds to the interface radius at 30 nm, the red at 20 nm, and the green at 10 nm. Distributions are calculated at θ e using models with volumetric ( ɛ t 0 ) (dotted line) and uniaxial ( ɛ tr ) (dashed line) transformation strains, as well as with equal thermoelastic properties of solid and melt (solid line), that is, for liquid–liquid transformation. Dots designate pressures in melt p s +2 γ s−l / r i based on the Laplace equation that coincides with results of calculations for equal thermoelastic properties of the solid and melt. Full size image Interface profile and energy For plane interface, θ = θ e , and neglected mechanics, the GL equation allows analytical solution for an equilibrium interface: where the interface width is δ =| r l − r s | and r l and r s are determined from the conditions φ ( η )=0.01 and 0.99, respectively. Surface energy in non-equilibrium state is defined as an excess energy with respect to solid (where 0.5< η ≤1) and liquid (where 0≤ η ≤0.5) With neglected mechanics, interface width is described by equation (9) within 2.5% error for r i ≥2 δ e and θ ≤1.25 θ e , that is, even above θ i . For r i =2 nm, δ =3.99 nm=1.34 δ e . Mechanics slightly (<1%) increases the width for θ = θ e , but this difference grows with increasing temperature; for example, δ =3.03 and 3.06 nm for r i =30 nm, θ =1.2 θ e and 1.25 θ e , respectively. Still, the interface profile differs from equation (9) within Δ φ =0.03 error for r i ≥ δ e /2 and θ ≤ θ i . 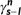Figure 7: Non-equilibrium interface energyversus interface radius for different temperatures. Results are obtained for both volumetric and uniaxial transformation strains and practically coincide. At the position ofri=10 nm, curves from top to bottom correspond to temperatures of 1.2θe, 1.1θe,θe, 0.9θeand 0.8θe. A crossover in temperature dependence of interface energy for radii below 20 nm is evident. Interface energy versus interface radius for different temperatures is shown in Figure 7 . For equilibrium temperature, interface energy starts growing for r i <10 nm and maximum deviation from γ s−l =0.1 J m −2 is 11.2% for the smallest r i =2.41 nm, for which full interface exists. For r i >20 nm expected decrease in with growing temperature is observed. For r i <20 nm, unexpectedly the opposite relation is found, which means change in sign of the interface entropy. Note that for r i >4 δ e ≃ 12 nm, deviation of from γ s−l does not exceed 3% in the entire temperature range θ c < θ < θ i , which is well below the inaccuracy of experimental data for interface energy. Figure 7: Non-equilibrium interface energy versus interface radius for different temperatures. Results are obtained for both volumetric and uniaxial transformation strains and practically coincide. At the position of r i =10 nm, curves from top to bottom correspond to temperatures of 1.2 θ e , 1.1 θ e , θ e , 0.9 θ e and 0.8 θ e . A crossover in temperature dependence of interface energy for radii below 20 nm is evident. 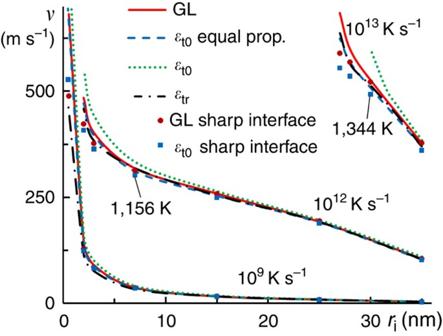Figure 8: Interface velocity versus position for three heating rates. The heating rate is 109K s−1at the bottom, 1012K s−1in the middle, and 1013K s−1at the top. Curves correspond to PFA with different models (red line for GL model, green and black lines for models with volumetric and uniaxial transformation strains, respectively, and blue line for volumetric transformation strain with equal solid and melt properties). Points correspond to SIA, namely, to equation (11). Full size image Interface velocity When internal stresses inside an interface are neglected, the following linear relationship is obtained for r i ≫ δ e between interface velocity v 0 and the thermodynamic force for interface propagation per unit deformed volume of solid X : It can be seen from Figure 8 that equation (11) describes well (error ≤3%) results of our simulations even for r i >2 δ e for neglected internal stresses and for heating rates as high as 10 13 K s −1 . Owing to small particle size, homogeneous temperature is assumed; see the analytical justification in ref. 8 . The temperature at some points in Figure 8 significantly exceeds the instability temperature θ i and reaches 1344 K for 10 13 K s −1 ; that is why interface does not reach the centre of the particle, because homogeneous reduction of η in the central part completes melting faster. Even for high compressive and tensile pressures, equation (11) works well when internal stresses are negligible: for external pressure p =4 GPa and θ =1225 K deviations from simulations for r i =30 and 20 nm are within 2.14%, and for p =−4 GPa and θ =750 K it is within 1.05%. Velocities for volumetric ɛ t are higher, and for uniaxial ɛ t they are lower than for the case with μ =0. Figure 8: Interface velocity versus position for three heating rates. The heating rate is 10 9 K s −1 at the bottom, 10 12 K s −1 in the middle, and 10 13 K s −1 at the top. Curves correspond to PFA with different models (red line for GL model, green and black lines for models with volumetric and uniaxial transformation strains, respectively, and blue line for volumetric transformation strain with equal solid and melt properties). Points correspond to SIA, namely, to equation (11). Full size image Note that the SIA [21] to melting/solidification at the nanoscale, which includes surface-induced melting and coupled to mechanics, can be applied to our problems down to some radius, which is to be determined by comparison with PFA. However, when the interface region is a significant part of the particle, PFA is more precise and does not require any adjustments. In contrast, SIA should incorporate the size dependence of surface melting ( Fig. 3 ), size and temperature dependence of surface energy ( Fig. 7 ), and surface stresses not equal to surface tension ( Fig. 6 ). To summarize, an advanced phase-field approach to premelting and melting coupled to mechanics is developed. It is applied to study melting deeply in the region of metastability and complete instability of solid and melt, intermediate states at the surface and in few nm-size particles, scale effect, and non-equilibrium thermodynamic and kinetic properties. The importance of mechanics effects (even without external pressure) is elucidated. Crossover in temperature dependence of the interface energy for radii below 20 nm and violation of the Laplace relationship for the jump in pressure is obtained. Conceptual validity of the coherent solid melt is proven and necessity for its further development, namely, formulation of the evolution equation for the deviatoric part of ɛ t , is demonstrated. The finite element method code COMSOL Multiphysics was utilized to solve coupled equations (2), (3), (4), (5), (6), (7), (8). Quadratic Lagrangian elements are used for both the mechanical and GL differential equations. In all, 15–30 elements per interface width and an adaptive time step with a minimum of 1,000 time steps for a typical non-stationary problem are used. To check the model, interface profiles are compared with analytical results for plane interface at equilibrium temperature [22] . Even with an interface radius of 30 nm, difference between planar analytical solution and COMSOL GL result is less than 0.1%. Also, the solid–liquid interface energy in Al practically coincides with its analytical value of 0.1 J m −2 , see Figure 7 . How to cite this article: Levitas, V.I. & Samani. K. Size and mechanics effects in surface-induced melting of nanoparticles. Nat. Commun. 2:284 doi: 10.1038/ncomms1275 (2011).